ArabidopsisERF109 mediates cross-talk between jasmonic acid and auxin biosynthesis during lateral root formation Jasmonic acid (JA) is well known to promote lateral root formation but the mechanisms by which JA signalling is integrated into the pathways responsible for lateral root formation, and how it interacts with auxin in this process remains poorly understood. Here, we report that the highly JA-responsive ethylene response factor 109 (ERF109) mediates cross-talk between JA signalling and auxin biosynthesis to regulate lateral root formation in Arabidopsis . erf109 mutants have fewer lateral roots under MeJA treatments compared with wild type whereas ERF109 overexpression causes a root phenotype that resembles those of auxin overproduction mutants. ERF109 binds directly to GCC-boxes in the promoters of ASA1 and YUC2 , which encode two key enzymes in auxin biosynthesis. Thus, our study reveals a molecular mechanism for JA and auxin cross-talk during JA-induced lateral root formation. Improved root architecture is crucial for crop productivity and a very important contributor to drought resistance [1] . Most dicotyledonous plants have tap root systems, whereas monocotyledonous plants have fibrous root systems composed of adventitious roots (AR) [2] . Primary root (PR) development starts during embryogenesis. Lateral root (LR) development is initiated from asymmetric divisions of the pericycle founder cell of PR and the whole process of development has been well established [3] , [4] . It is well known that the phytohormone auxin has a very important role in root development [5] . It is involved in every stage of LR formation [5] , [6] . Auxin biosynthesis, transport and auxin-dependent signalling processes all affect LR formation [7] , [8] , [9] . In Arabidopsis roots, an elevated auxin level causes the degradation of indole-3-acetic acid/auxin (IAA/AUX) and increases the levels of auxin response factors (ARFs) [10] , [11] . ARFs activate the functions of lateral organ boundaries-domain (LBD) to promote LR formation and enhance LR density [12] , [13] . Mutations in the genes involved in auxin biosynthesis, transport and signalling greatly impact LR initiation and formation [3] , [6] . Auxin overproduction mutants, such as the gain-of-function yucca mutant, superroot1 ( sur1 ), sur2 and arf8 , increase LR number [3] , [14] . The mutants with defects in auxin transport, such as auxin resistant 1 ( aux1 ), like aux1 3 ( lax3 ), pin-formed ( pin ) multiple mutants, gnom and auxin resistant 4 ( axr4 ), have reduced LR number or aberrant lateral root primodium (LRP) [3] . Auxin signalling mutants, including arf7 arf19 double mutants, gain-of-function iaa14 / solitaryroot 1 ( slr1 ) mutant, gain-of-function iaa19/ massugu 2 ( msg2 ) mutant, gain-of-function iaa28 mutant and lbd16 lbd18 double mutants, show severe damage or complete absence of LR formation [3] , [5] . Interactions among plant hormones form a complex network to regulate developmental processes [15] , [16] . In most cases, other hormones regulate root development through the interaction with auxin [6] , [17] . Among these hormones, the functions of jasmonic acid (JA) in wounding and defence responses of plants were well studied and its roles in plant growth and development were also reported [18] , [19] . With exogenous JA treatments, plants showed short PRs and more LRs [20] . Interactions of JA with other hormones have been reported [21] . JA and auxin share some signalling pathway components [22] , [23] , [24] . These two plant hormones have demonstrated cross-talk through the action of ARFs [25] . In addition, JA signalling pathway is linked to auxin homeostasis through the modulation of YUCCA8 ( YUC8 ) and YUC9 gene expressions [26] , [27] . Anthranilate synthase alpha subunit 1 ( ASA1 , At5g05730), which encodes an L-tryptophan (Trp) biosynthesis enzyme, mediates JA-induced auxin accumulation and transport [28] . The transcription levels of several genes involved in auxin biosynthesis are also upregulated by methyl jasmonate (MeJA) [28] . Among these genes, YUC2 (At4g13260) encodes a flavin monooxygenase-like enzyme, which catalyses a rate-limiting step in Trp-dependent auxin biosynthesis pathway with functional redundancy of YUCCA family [14] , [29] . Furthermore, JA was reported to affect auxin transport [30] . Despite the recent progress, the molecular mechanisms underlying the interaction between JA and IAA are far from being well understood. The Arabidopsis mutant enhanced drought tolerance 1 ( edt1 ) showed improved drought tolerance with a more extensive root system, which was caused by the strong expression of the homeodomain transcription factor homeodomain glabrous 11 ( HDG11 ) in a constitutive fashion [31] . To study the molecular mechanisms of improved root architecture of edt1 , the root transcriptomes of edt1 and the wild type were compared. We found that a transcription factor named ethylene response factor 109 ( ERF109) (At4g34410) was remarkably upregulated in the roots of edt1 seedlings. ERF109 encodes a plant specific transcription factor of the ERF family, which contains only one APETALA2 (AP2) domain responsible for binding to the promoters of downstream target genes [32] , [33] , [34] . ERFs are also named as ethylene-responsive element binding proteins (EREBPs), which were first identified in tobacco and found to directly bind to the cis -element called a GCC-box containing the core 5′- GCCGCC -3′ sequence [32] . The transcription of ERF109 is inducible by MeJA treatment [35] . In addition, ERF109 was reportedly expressed during the re-adjustment of Arabidopsis leaves to homeostasis after high light stress, and consequently named redox-responsive transcription factor 1 (ref. 36 ). Here, we report that AtERF109 integrates JA signalling into auxin pathways to regulate root architecture. Although it is very weakly expressed under normal growth conditions, ERF109 is highly responsive to MeJA treatment in Arabidopsis roots. Genetic analysis with ERF109 knockout mutants and overexpression lines demonstrates that ERF109 regulates LRP development and JA-induced LR formation. The ERF109 overexpression lines (35S- ERF109 ) show shorter PR, increased number of LRP, enhanced LR density and other phenotypes typical of those caused by elevated auxin levels. We also find that ERF109 binds directly to the promoters of ASA1 and YUC2 , which encode key enzymes in auxin biosynthesis pathways. ERF109 is highly responsive to MeJA JA-induced expression of ERF109 was analysed in a time course. ERF109 was transiently upregulated by MeJA treatments. The transcript level of ERF109 peaked with a 20-fold induction at 20 min and was restored to the previous level at 1 h after MeJA treatment, which is in agreement with the previous report ( Fig. 1a ) [35] . 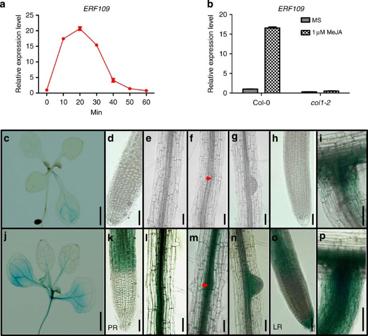Figure 1:ERF109is highly responsive to MeJA. (a)ERF109is transiently induced by MeJA. The time course analysis ofERF109expression in response to MeJA treatment was conducted. Col-0 seedlings were grown on MS medium vertically for 14 days. Then, the seedlings were transferred to MS medium without (control) or with 1 μM MeJA for the indicated times before RNA extraction. RNA was isolated at indicated time points and quantitative RT–PCR analysis was performed subsequently. Values are mean±s.d. (n=3 experiments). (b) MeJA-induced expression ofERF109requires the function of COI1. The 14-day-old Col-0 andcoi1-2seedlings were treated with 1 μM of MeJA for 0.5 h. Then RNA was isolated and quantitative RT–PCR analysis was performed. Values are mean±s.d. (n=3 experiments). (c–i) GUS staining of 7-day-old transgenic lines containedERF109pro-GUSwithout MeJA treatment. GUS expressions in cotyledon (c), primary root (d), stele (e), LRP at all developmental stages (fandg) and the tip and base of LR (handi). (c) Scale bar, 1 mm; (d–i) Scale bars, 50 μm. (j–p) GUS staining of 7-day-old transgenic lines containedERF109pro-GUSwith 10 μM MeJA treatment for 0.5 h. GUS expressions were significantly enhanced in cotyledon (j), primary root (k), stele (l), LRP at all developmental stages (mandn) and the tip and base of LR (oandp). (j) Scale bar, 1 mm; (k–p) Scale bars, 50 μm.The locations of LRPs are shown by red arrows infandm. Figure 1: ERF109 is highly responsive to MeJA. ( a ) ERF109 is transiently induced by MeJA. The time course analysis of ERF109 expression in response to MeJA treatment was conducted. Col-0 seedlings were grown on MS medium vertically for 14 days. Then, the seedlings were transferred to MS medium without (control) or with 1 μM MeJA for the indicated times before RNA extraction. RNA was isolated at indicated time points and quantitative RT–PCR analysis was performed subsequently. Values are mean±s.d. ( n =3 experiments). ( b ) MeJA-induced expression of ERF109 requires the function of COI1. The 14-day-old Col-0 and coi1-2 seedlings were treated with 1 μM of MeJA for 0.5 h. Then RNA was isolated and quantitative RT–PCR analysis was performed. Values are mean±s.d. ( n =3 experiments). ( c – i ) GUS staining of 7-day-old transgenic lines contained ERF109pro-GUS without MeJA treatment. GUS expressions in cotyledon ( c ), primary root ( d ), stele ( e ), LRP at all developmental stages ( f and g ) and the tip and base of LR ( h and i ). ( c ) Scale bar, 1 mm; ( d – i ) Scale bars, 50 μm. ( j – p ) GUS staining of 7-day-old transgenic lines contained ERF109pro-GUS with 10 μM MeJA treatment for 0.5 h. GUS expressions were significantly enhanced in cotyledon ( j ), primary root ( k ), stele ( l ), LRP at all developmental stages ( m and n ) and the tip and base of LR ( o and p ). ( j ) Scale bar, 1 mm; ( k – p ) Scale bars, 50 μm.The locations of LRPs are shown by red arrows in f and m . Full size image The responses of ERF109 to different hormones and stresses were analysed using β-glucuronidase (GUS) staining and quantitative PCR with reverse transcription (RT–PCR) subsequently ( Supplementary Fig. 1 ). The GUS staining was significantly induced by MeJA and weakly induced by salicylic acid (SA) and 1-aminocyclopropane-1-carboxylic acid (ACC) ( Supplementary Fig. 1a–d ), but apparently not by abscisic acid (ABA), gibberellin (GA), IAA or 6-benzylaminopurine (6-BA) treatments ( Supplementary Fig. 1e–h ). Interestingly, the expression of ERF109 was also weakly induced by NaCl and paraquat (PQ) treatments ( Supplementary Fig. 1i,k ). The quantitative RT–PCR results are consistent with the GUS staining for MeJA, SA, ACC, IAA, 6-BA, NaCl, mannitol and PQ treatments, but not for ABA and GA that slightly induced the expression of ERF109 ( Supplementary Fig. 1l ). In addition, no significant difference was found during the salt-induced adventitious root formation ( Supplementary Fig. 1m–o ). Under normal conditions, ERF109 was expressed in all tissues examined but at low levels in roots as demonstrated by quantitative RT–PCR and ERF109pro-GUS reporter analyses ( Supplementary Fig. 2 ). However, in the coronatine insensitive 1 ( coi1 ) background, MeJA-induced expression of ERF109 was abolished, which is in agreement with a previous report ( Fig. 1b ) [35] . This result indicates that MeJA-induction of ERF109 requires the function of COI1, the receptor of JA-isoleucine (Ile) in Arabidopsis [35] , [37] , [38] , [39] . Therefore, ERF109 is under the regulation of JA signalling. To study the spatial pattern of ERF109 in response to JA treatments, we treated the ERF109pro-GUS reporter lines with MeJA for 0.5 h. The GUS staining results showed that under normal conditions, ERF109 was very weakly expressed only in the tip and base of LRs in the roots ( Fig. 1c–i ). However, in response to MeJA treatment, the expression of ERF109 was dramatically induced in both shoots and roots, especially in the region behind PR tip, stele, LRP and the tip and base of LRs ( Fig. 1j–p ). As predicted for a transcription factor, ERF109 was localized in nuclei ( Supplementary Fig. 3 ). ERF109 regulates LR development in response to MeJA To study the function of ERF109 in root development, we identified a loss-of-function mutant erf109 and generated 35S- ERF109 transgenic lines ( Supplementary Fig. 4 ). The LRP of the wild-type (Col-0), erf109 and 35S- ERF109 lines were subsequently examined and quantified. In this study, LRP were counted on the basis of expression of the DR5-GUS marker gene. As shown in Fig. 2a,b , erf109 had fewer LRP per unit root length than wild type under normal conditions. In contrast, the number of LRP in 35S- ERF109 -1 was significantly increased. Similarly, we observed additional transgenic lines of 35S- ERF109 , which showed shorter PRs and more LRs than wild type ( Supplementary Fig. 5 ). 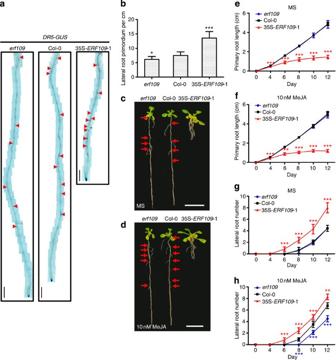Figure 2:ERF109regulates LRP development in response to MeJA. (a)erf109had fewer LRP and 35S-ERF109-1 had more LRP than the wild type. The locations of LRPs were indicated by red triangles. Scale bar, 0.5 mm. (b) The numbers of LRPs of 5-day-old wild-type,erf109and 35S-ERF109-1 seedlings were counted. Values are mean±s.d. (n=10 seedlings, *P<0.05, ***P<0.001). Asterisks indicate Student’st-test significant differences. (c,d) The root phenotypes of the wild-type,erf109and 35S-ERF109-1 seedlings grown on MS without (c) or with 10 nM MeJA (d). The locations of LRs were indicated by red arrows. Scale bar, 1 cm. (e,f) PR elongation of the wild-type,erf109and 35S-ERF109-1 seedlings grown on MS without (e) or with 10 nM MeJA (f) were measured at the indicated time points. Values are mean±s.d. (n=25 seedlings, ***P<0.001). Asterisks indicate Student’st-test significant differences. In (e–g), theerf109and Col-0 data overlap so heavily that they are difficult to distinguish. (g,h) The numbers of LRs of the wild-type,erf109and 35S-ERF109-1 seedlings grown on MS without (g) or with 10 nM MeJA (h) were counted at the indicated time points. Values are mean±s.d. (n=25 seedlings, ***P<0.001). Asterisks indicate Student’st-test significant differences. Figure 2: ERF109 regulates LRP development in response to MeJA. ( a ) erf109 had fewer LRP and 35S- ERF109 -1 had more LRP than the wild type. The locations of LRPs were indicated by red triangles. Scale bar, 0.5 mm. ( b ) The numbers of LRPs of 5-day-old wild-type, erf109 and 35S- ERF109 -1 seedlings were counted. Values are mean±s.d. ( n =10 seedlings, * P <0.05, *** P <0.001). Asterisks indicate Student’s t -test significant differences. ( c , d ) The root phenotypes of the wild-type, erf109 and 35S- ERF109 -1 seedlings grown on MS without ( c ) or with 10 nM MeJA ( d ). The locations of LRs were indicated by red arrows. Scale bar, 1 cm. ( e , f ) PR elongation of the wild-type, erf109 and 35S- ERF109 -1 seedlings grown on MS without ( e ) or with 10 nM MeJA ( f ) were measured at the indicated time points. Values are mean±s.d. ( n =25 seedlings, *** P <0.001). Asterisks indicate Student’s t -test significant differences. In ( e – g ), the erf109 and Col-0 data overlap so heavily that they are difficult to distinguish. ( g , h ) The numbers of LRs of the wild-type, erf109 and 35S- ERF109 -1 seedlings grown on MS without ( g ) or with 10 nM MeJA ( h ) were counted at the indicated time points. Values are mean±s.d. ( n =25 seedlings, *** P <0.001). Asterisks indicate Student’s t -test significant differences. Full size image To examine the response of roots to MeJA, we transferred 3-day-old seedlings to MS medium without or with MeJA and grown vertically. The PR length of erf109 was not different from that of wild type. However, the PR length of 35S- ERF109 -1 was significantly reduced ( Fig. 2c,e ). Treatment with 10 nM MeJA did not affect the PR length of erf109 , wild type and 35S- ERF109 -1 ( Fig. 2d,f ). We also included an asa1 mutant in the experiment and examined the dose response of erf109 , wild type, 35S- ERF109 -1, 35S -ERF109 -2 and asa1 for PR elongation at higher concentrations of MeJA. The erf109 , wild type and asa1 showed similar PR response to all tested concentrations of exogenous MeJA ( Supplementary Fig. 6 ). LR number in wild type, erf109 and 35S- ERF109 -1 grown on MS medium was also counted. The erf109 mutant had a similar number of LRs as wild type. However, 35S- ERF109 -1 had significantly more LRs ( Fig. 2c,g ). In response to 10 nM MeJA treatment, wild type showed increased number of LR but not erf109 ( Fig. 2d,h ). These results strongly indicate that ERF109 has a positive role in LR formation. We also examined MeJA dose response of erf109 , wild type, 35S- ERF109 -1, 35S- ERF109 -2 and asa1 for LR formation. The erf109 and asa1 mutants show less LR formation than wild type under a range dose of MeJA ( Supplementary Fig. 7 ). The phenotypes of erf109 , wild type and 35S- ERF109 -1 in response to salt stress were observed subsequently ( Supplementary Fig. 8 ). LR development was induced by salt treatment. This induction was reduced in erf109 under 150 mM salt treatment. To demonstrate whether the observed phenotypes were caused by ERF109 , erf109 was complemented by a 35S- ERF109 cDNA construct. A line with similar expression level of ERF109 to that in wild type was used to test for functional complementation (FC) and observation of LR formation ( Supplementary Fig. 9a ). Consistent with previous results, the erf109 had fewer LRP than wild type, while the number of LRP of FC (FC-27) was not different from that of wild type ( Supplementary Fig. 9b ). In addition, consistent with wild type, FC also showed increased LR formation in comparison with erf109 under 10 nM MeJA treatment ( Supplementary Fig. 9c,d ). To confirm this, we analysed additional FC lines with various expression levels of ERF109 and found that FC lines with high transgene expression showed similar phenotypes as the 35S- ERF109 ( Supplementary Fig. 10 ). These results further indicate that ERF109 has a positive role in LR formation. 35S- ERF109 lines show auxin overproduction phenotypes In addition to the short PRs and increased numbers of LRP and LR, 35S- ERF109 -1 and 35S- ERF109 -2 had other phenotypes typical of elevated auxin level, such as long hypocotyl, much longer and more root hair ( Fig. 3a–c ). Mature leaves of 35S- ERF109 -1 were longer, narrower and curled downward with longer petioles compared with those of the wild type ( Fig. 3d ). These phenotypes are similar to those caused by elevated auxin levels as previously reported [14] . These results suggest that ERF109 might upregulate auxin biosynthesis. 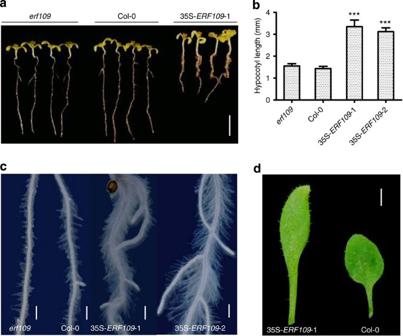Figure 3: Auxin overproduction phenotypes of 35S-ERF109plants. (a) 35S-ERF109-1 seedlings had longer hypocotyls than wild type. Scale bar, 0.5 cm. (b) Hypocotyl elongation of the wild-type,erf10935S-ERF109-1 and 35S-ERF109-2 seedlings grown on MS were measured at the indicated time points. Values are mean±s.d. (n=10 seedlings, ***P<0.001). Asterisks indicate Student’st-test significant differences. (c) Root hair of the wild-type,erf109, 35S-ERF109-1and 35S-ERF109-2seedlings. Scale bar, 0.5 mm. (d) Mature leaves of the wild-type and 35S-ERF109-1 seedlings. Scale bar, 2 mm. Figure 3: Auxin overproduction phenotypes of 35S- ERF109 plants. ( a ) 35S- ERF109 -1 seedlings had longer hypocotyls than wild type. Scale bar, 0.5 cm. ( b ) Hypocotyl elongation of the wild-type, erf109 35S- ERF109 -1 and 35S- ERF109 -2 seedlings grown on MS were measured at the indicated time points. Values are mean±s.d. ( n =10 seedlings, *** P <0.001). Asterisks indicate Student’s t -test significant differences. ( c ) Root hair of the wild-type, erf109 , 35S- ERF109-1 and 35S- ERF109-2 seedlings. Scale bar, 0.5 mm. ( d ) Mature leaves of the wild-type and 35S- ERF109 -1 seedlings. Scale bar, 2 mm. Full size image ERF109 elevates auxin level To investigate whether ERF109 indeed upregulates auxin level, we measured endogenous free IAA contents with liquid chromatography–tandem mass spectrometry system in wild-type, erf109 and 35S- ERF109 -1 seedlings. As shown in Fig. 4a , auxin levels in the shoot and root tissues of erf109 were reduced compared with that of the wild type. In contrast, 35S- ERF109 -1 had significantly higher auxin levels in both shoot and root tissues than the wild type. Consistent with these results, the expression of the marker genes involved in auxin-dependent signalling processes related to LR development was also affected ( Fig. 4b–d ). The expressions of IAA14 (At4g14550) and IAA19 (At3g15540) were downregulated in the shoot tissue of 35S- ERF109 -1. The erf109 had lower levels of LBD16 (At2g42430) transcript in both shoot and root tissues than wild type, while the opposite results were observed in 35S- ERF109 -1. The altered expression of these genes was consistent with the root phenotypes and auxin levels of wild type, erf109 and 35S- ERF109 . JA-induced ERF109 enhanced auxin biosynthesis to regulate Arabidopsis root architecture. 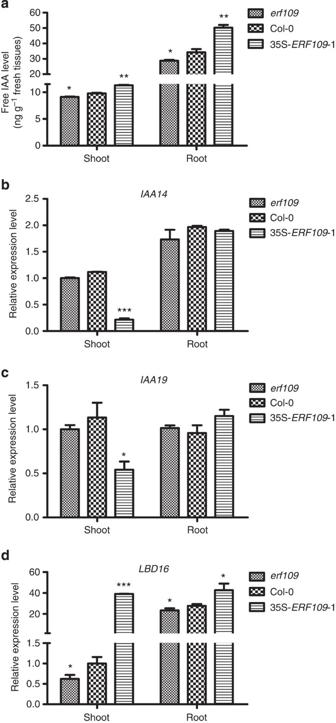Figure 4:ERF109elevates auxin level inArabidopsis. (a) Free IAA concentration in shoot and root of the wild-type,erf109and 35S-ERF109-1 seedlings. Two-week-old seedlings were divided into shoots and roots for IAA measurements using LC-MS. Values are mean±s.e. (four biological repeats, *P<0.05, **P<0.01). Asterisks indicate Student’st-test significant differences. (b–d) Quantitative RT–PCR analysis of the marker genes involved in auxin-dependent signalling processes. RNA was isolated from the shoots and roots of two-week-old seedlings of the wild-type,erf109and 35S-ERF109-1. Values are mean±s.d. (n=3 experiments, *P<0.05, ***P<0.001). Asterisks indicate Student’st-test significant differences. Figure 4: ERF109 elevates auxin level in Arabidopsis . ( a ) Free IAA concentration in shoot and root of the wild-type, erf109 and 35S- ERF109 -1 seedlings. Two-week-old seedlings were divided into shoots and roots for IAA measurements using LC-MS. Values are mean±s.e. (four biological repeats, * P <0.05, ** P <0.01). Asterisks indicate Student’s t -test significant differences. ( b – d ) Quantitative RT–PCR analysis of the marker genes involved in auxin-dependent signalling processes. RNA was isolated from the shoots and roots of two-week-old seedlings of the wild-type, erf109 and 35S- ERF109 -1. Values are mean±s.d. ( n =3 experiments, * P <0.05, *** P <0.001). Asterisks indicate Student’s t -test significant differences. Full size image DR5-GUS reporter was introduced into wild type, erf109 and 35S- ERF109 -1 backgrounds. In the erf109 background, GUS staining in shoot tissue was weaker than that in wild type. In contrast, the shoot tissue of 35S- ERF109 -1 was strongly stained as compared with wild type ( Fig. 5a ). In root tissues, DR5-GUS expression in PR tips was weaker in erf109 and stronger in 35S- ERF109 -1 than that of wild type ( Fig. 5a ). 35S- ERF109 -1 also had elevated expression levels of DR5-GUS in the LRPs at different developmental stages and the LR tips as compared with wild type, while erf109 had lower levels than wild type ( Fig. 5b ). 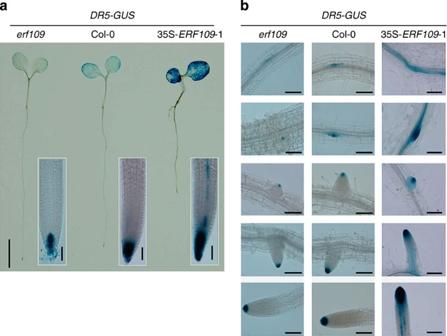Figure 5: Altered expression ofDR5-GUSmarker in variedERF109backgrounds. (a)DR5-GUSexpression levels in 5-day-olderf109, wild-type and 35S-ERF109-1 seedlings. Scale bar, 0.2 cm.DR5-GUSexpression levels in the PR tipsof7-day-olderf109, wild type and 35S-ERF109-1 seedlings were shown next to the seedlings. Scale bar, 50 μm. (b) The comparison ofDR5-GUSexpression levels in the initiation sites of LRP, LRPs and LR tips between two-week-olderf109, wild type and 35S-ERF109-1. Scale bar, 100 μm. Figure 5: Altered expression of DR5-GUS marker in varied ERF109 backgrounds. ( a ) DR5-GUS expression levels in 5-day-old erf109 , wild-type and 35S- ERF109 -1 seedlings. Scale bar, 0.2 cm. DR5-GUS expression levels in the PR tips of 7-day-old erf109 , wild type and 35S- ERF109 -1 seedlings were shown next to the seedlings. Scale bar, 50 μm. ( b ) The comparison of DR5-GUS expression levels in the initiation sites of LRP, LRPs and LR tips between two-week-old erf109 , wild type and 35S- ERF109 -1. Scale bar, 100 μm. Full size image ERF109 regulates the transcription of ASA1 and YUC2 To identify downstream targets of ERF109, we searched for GCC-boxes in the promoters of auxin biosynthesis and transport genes and found that both ASA1 and YUC2 contained one GCC-box in their promoters. To find out whether ERF109 can directly activate the transcriptions of ASA1 and YUC2 , we first performed quantitative RT–PCR analysis using wild type, erf109 and 35S- ERF109 -1 seedlings divided into shoot and root tissues. The data showed that both the candidate target genes could be downregulated in the shoot and root tissues of erf109 and upregulated in 35S- ERF109 -1 ( Fig. 6a ). 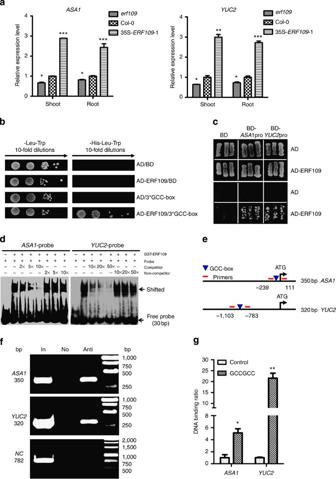Figure 6: ERF109 directly regulates the transcriptions ofASA1andYUC2. (a) Quantitative RT–PCR analysis of transcriptions ofASA1andYUC2. The shoots and roots of two-week-olderf109, wild-type and 35S-ERF109-1 seedlings were used. Values are mean±s.d. (n=3 experiments, **P<0.01, ***P<0.001). Asterisks indicate Student’st-test significant differences. (b) Yeast-one-hybrid assay for ERF109 binding to the fragment containing three copies of core sequence of GCC-box in tandem repeat. A serial yeast dilutions (1:1, 1:10, 1:100 and 1:1,000) were grown on SD medium lacking Leu and Trp, and the same medium lacking Leu, Trp and His. The empty pAD and pHIS2 vectors were used as negative control. (c) Yeast-one-hybrid assay for ERF109 binding to two 30 bp sequences containing the GCC-boxes from the promoter ofASA1orYUC2, respectively. The six panels on the top showed that yeast were grown on SD medium (-Leu-Trp), and the six panels on the bottom indicated that yeast were grown on SD medium (-His-Leu-Trp). (d) EMSA. Unlabelled probes were used as competitors and mutated probes were used as non-competitors. ERF109-dependent mobility shifts were detected and unlabelled probe competed in a dose-dependent manner while the non-competitor probe did not. (e) The schematic illustration of the locations of GCC-boxes (inverted triangles) in the promoters ofASA1andYUC2and the primers used for RT–PCR and quantitative RT–PCR (short lines). (f,g). ChIP assay. About 300 bpASA1andYUC2promoter fragments containing GCC-boxes were enriched by anti-HA antibodies in RT–PCR analysis (f). The region oftubulin8(TUB8, At5g23860) that do not contain a GCC-box was used as a negative control. In (Input), the chromatin DNA was used as the template; No, ChIP with no antibody was used as the template for negative control; Anti, ChIP with anti-HA antibody was used as the template. M, DNA size marker. The results of ChIP–PCR were confirmed by quantitative RT–PCR (g). The regions ofASA1andYUC2that do not contain GCC-box were used as negative controls. Values are mean±s.d. (n=3 experiments, *P<0.05, **P<0.01). Asterisks indicate Student’st-test significant differences. Figure 6: ERF109 directly regulates the transcriptions of ASA1 and YUC2 . ( a ) Quantitative RT–PCR analysis of transcriptions of ASA1 and YUC2 . The shoots and roots of two-week-old erf109 , wild-type and 35S- ERF109 -1 seedlings were used. Values are mean±s.d. ( n =3 experiments, ** P <0.01, *** P <0.001). Asterisks indicate Student’s t -test significant differences. ( b ) Yeast-one-hybrid assay for ERF109 binding to the fragment containing three copies of core sequence of GCC-box in tandem repeat. A serial yeast dilutions (1:1, 1:10, 1:100 and 1:1,000) were grown on SD medium lacking Leu and Trp, and the same medium lacking Leu, Trp and His. The empty pAD and pHIS2 vectors were used as negative control. ( c ) Yeast-one-hybrid assay for ERF109 binding to two 30 bp sequences containing the GCC-boxes from the promoter of ASA1 or YUC2 , respectively. The six panels on the top showed that yeast were grown on SD medium (-Leu-Trp), and the six panels on the bottom indicated that yeast were grown on SD medium (-His-Leu-Trp). ( d ) EMSA. Unlabelled probes were used as competitors and mutated probes were used as non-competitors. ERF109-dependent mobility shifts were detected and unlabelled probe competed in a dose-dependent manner while the non-competitor probe did not. ( e ) The schematic illustration of the locations of GCC-boxes (inverted triangles) in the promoters of ASA1 and YUC2 and the primers used for RT–PCR and quantitative RT–PCR (short lines). ( f , g ). ChIP assay. About 300 bp ASA1 and YUC2 promoter fragments containing GCC-boxes were enriched by anti-HA antibodies in RT–PCR analysis ( f ). The region of tubulin8 ( TUB8 , At5g23860) that do not contain a GCC-box was used as a negative control. In (Input), the chromatin DNA was used as the template; No, ChIP with no antibody was used as the template for negative control; Anti, ChIP with anti-HA antibody was used as the template. M, DNA size marker. The results of ChIP–PCR were confirmed by quantitative RT–PCR ( g ). The regions of ASA1 and YUC2 that do not contain GCC-box were used as negative controls. Values are mean±s.d. ( n =3 experiments, * P <0.05, ** P <0.01). Asterisks indicate Student’s t -test significant differences. Full size image Subsequently, we conducted yeast-one-hybrid assay to determine if ERF109 could directly bind to the GCC-boxes in the promoters of ASA1 and YUC2 . The results showed that ERF109 was able to bind to the GCC-boxes in the promoters of ASA1 and YUC2 in yeast cells ( Fig. 6b,c ). To determine whether ERF109 can directly bind in vitro to the GCC-boxes in the promoters of ASA1 and YUC2 , we conducted electrophoretic mobility shift assay (EMSA) with GST–ERF109 fusion protein expressed in E. coli . As shown in Fig. 6d , the GST–ERF109 fusion protein was able to directly bind to the DNA probes containing the 5′- GCCGCC -3′ motif as in the ASA1 and YUC2 promoters. The binding was specific as demonstrated by competition assay using unlabelled (competitor) and mutated probes (non-competitor). To confirm whether the interaction between ERF109 and the GCC-boxes of ASA1 and YUC2 promoters takes place in vivo , we performed chromatin immunoprecipitation (ChIP) assays using the transgenic plants expressing 35S-haemagglutinin (HA) -ERF109 with similar phenotypes to 35S- ERF109 plants and anti-HA antibodies. As shown in Fig. 6e–g , the ASA1 and YUC2 promoter regions containing the GCC-boxes were significantly enriched by ERF109. Thus, the specific binding of ERF109 to the GCC-boxes in the promoters of ASA1 and YUC2 was confirmed in Arabidopsis . To visualize the altered spatiotemporal expression patterns of ASA1 and YUC2 by ERF109 in Arabidopsis , the ASA1pro-GUS and YUC2pro-GUS reporters were introduced into wild type, erf109 and 35S- ERF109 -1 background by crossing. We first examined the response of ASA1pro-GUS and YUC2pro-GUS reporter to MeJA treatment in different ERF109 background. Without exogenous MeJA treatment, the expression level of ASA1 and YUC2 was slightly lower in the root tissues of erf109 than that in wild type. In response to 10 nM MeJA treatment for 0.5 h, the expression of ASA1 and YUC2 was elevated in the root of the wild type. However, it was not affected in erf109 root under the same MeJA treatment ( Fig. 7a,b ). In the 35S- ERF109 -1 background, the expression of ASA1 and YUC2 did not show significant difference to MeJA treatment due to the high level expression of ERF109 from the 35S promoter, which likely overshadowed the JA-induced expression of ERF109 . 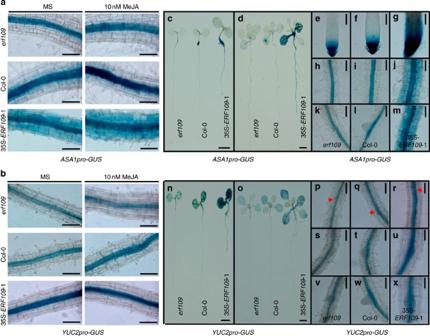Figure 7: Altered expression ofASA1pro-GUSandYUC2pro-GUSin variedERF109genetic backgrounds. (a,b) The expression of eitherASA1pro-GUSorYUC2 pro-GUScould not be induced by 10 nM MeJA treatment for 0.5 h inerf109compared with that in the wild-type. 7-day-old seedlings were transferred to MS without or with 10 nM MeJA for 0.5 h before GUS staining. Scale bar, 100 μm. (c–m) The expression levels ofASA1pro-GUSin both the shoot and root tissues oferf109, wild type and 35S-ERF109-1. The GUS staining in the shoot tissues were observed using 5-day-old (c) and 10-day-old seedlings (d). Scale bar, 0.2 cm. The GUS staining in the PR tip (e–g), stele of maturation zone (h–j) and the LRP (k–m) were observed using 7-day-olderf109, wild-type and 35S-ERF109-1 seedlings. Scale bar, 100 μm. (n–x) The expression levels ofYUC2pro-GUSin both the shoot and root tissues oferf109, wild type and 35S-ERF109-1. The expression levels ofYUC2pro-GUSin the shoot tissues were observed using 5-day-old (n) and 10-day-old seedlings (o). Scale bar, 0.2 cm. The expressions ofYUC2pro-GUSin the root tissues of 7-day-olderf109, wild type and 35S-ERF109-1 were observed (p–x). GUS staining was compared in the stele of maturation zone with LRP at the same developmental stages (early LRP,p–r, the locations of LRPs were shown using red arrows; middle LRP,s–u; and late LRP,v–x). Scale bar, 100 μm. Figure 7: Altered expression of ASA1pro-GUS and YUC2pro-GUS in varied ERF109 genetic backgrounds. ( a , b ) The expression of either ASA1pro-GUS or YUC2 pro-GUS could not be induced by 10 nM MeJA treatment for 0.5 h in erf109 compared with that in the wild-type. 7-day-old seedlings were transferred to MS without or with 10 nM MeJA for 0.5 h before GUS staining. Scale bar, 100 μm. ( c – m ) The expression levels of ASA1pro-GUS in both the shoot and root tissues of erf109 , wild type and 35S- ERF109 -1. The GUS staining in the shoot tissues were observed using 5-day-old ( c ) and 10-day-old seedlings ( d ). Scale bar, 0.2 cm. The GUS staining in the PR tip ( e – g ), stele of maturation zone ( h – j ) and the LRP ( k – m ) were observed using 7-day-old erf109 , wild-type and 35S- ERF109 -1 seedlings. Scale bar, 100 μm. ( n – x ) The expression levels of YUC2pro-GUS in both the shoot and root tissues of erf109 , wild type and 35S- ERF109 -1. The expression levels of YUC2pro-GUS in the shoot tissues were observed using 5-day-old ( n ) and 10-day-old seedlings ( o ). Scale bar, 0.2 cm. The expressions of YUC2pro-GUS in the root tissues of 7-day-old erf109 , wild type and 35S- ERF109 -1 were observed ( p – x ). GUS staining was compared in the stele of maturation zone with LRP at the same developmental stages (early LRP, p – r , the locations of LRPs were shown using red arrows; middle LRP, s – u ; and late LRP, v – x ). Scale bar, 100 μm. Full size image We then examined the expression of ASA1pro-GUS and YUC2pro-GUS reporter in different tissues in different ERF109 background. Either in 5- or 10-day-old seedlings, ASA1pro-GUS reporter was highly activated in cotyledons and roots in 35S- ERF109 -1 background compared with that in the wild type ( Fig. 7c,d ). In erf109 background, its expression level was slightly lower than that in the wild type ( Fig. 7c,d ). This was more evident in the closer examination of root tip ( Fig. 7e–g ), maturation zone ( Fig. 7h–j ) and the region with LRP ( Fig. 7k–m ). The higher expression level of ASA1pro-GUS was observed in the root tips and stele in 35S- ERF109 -1 background and the lowest level in erf109 background ( Fig. 7e–m ). The expression of YUC2pro-GUS reporter was very similar to that of ASA1pro-GUS ( Fig. 7n–x ) except that GUS staining was hardly visible in the root tips. The GUS staining results also showed that ERF109 , ASA1 and YUC2 had common expression patterns ( Figs 1 and 7 and Supplementary Fig. 2 ). The results agree with the binding between ERF109 and the GCC-box in the promoters of ASA1 and YUC2 . To confirm further that YUC2 is the target of ERF109, we introduced 35S- ERF109 into yuc2 mutant background by crossing 35S- ERF109 -1 with yuc2 . The genetic assay showed that the root phenotype of 35S- ERF109 -1 yuc2 was intermediate between 35S- ERF109 -1 and yuc2 ( Fig. 8 ), which demonstrates that YUC2 is one of the targets of ERF109 and suggests that ERF109 also affects PR length and LR number through other unidentified targets. 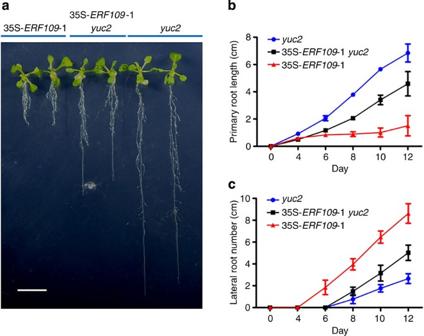Figure 8:YUC2acts downstream of ERF109. (a) The root phenotypes of 35S-ERF109-1, 35S-ERF109-1yuc2andyuc2seedlings grown on MS. Scale bar, 1 cm. (b) PR elongation of 35S-ERF109-1, 35S-ERF109-1yuc2andyuc2grown on MS were measured at the indicated time points. Values are mean±s.d. (n=15 seedlings). (c) The numbers of LRs of 35S-ERF109-1, 35S-ERF109-1yuc2andyuc2seedlings grown on MS were counted at the indicated time points. Values are mean±s.d. (n=15 seedlings). Figure 8: YUC2 acts downstream of ERF109. ( a ) The root phenotypes of 35S- ERF109 -1, 35S- ERF109 -1 yuc2 and yuc2 seedlings grown on MS. Scale bar, 1 cm. ( b ) PR elongation of 35S- ERF109 -1, 35S- ERF109 -1 yuc2 and yuc2 grown on MS were measured at the indicated time points. Values are mean±s.d. ( n =15 seedlings). ( c ) The numbers of LRs of 35S- ERF109 -1, 35S- ERF109 -1 yuc2 and yuc2 seedlings grown on MS were counted at the indicated time points. Values are mean±s.d. ( n =15 seedlings). Full size image It is well known that exogenous application of JA dramatically alters root system architecture. Yet the mechanism by which endogenous JA regulates root development remains poorly understood. An endogenous hormone, JA can be generated in response to various environmental stimuli. JA production can also be induced by ectopic expression of transcriptional regulators such as EDT1/HDG11 that activate JA biosynthesis genes, contributing to an improved root system [31] , [40] . JA is known to activate several types of transcription factors and mediate different responses to biotic and abiotic stresses. A number of transcription factors involved in JA signalling, plant defence and wounding response were identified via genome-wide screen and microarray analysis [35] , [41] . Transcription factors that respond to JA belong to several large gene families, including ERF, basic Leucine Zipper (bZIP), MYB, MYC and WRKY families [42] . MYC transcription factors are conserved in dicotyledonous plants, and have an important role in JA-mediated regulation of defence and wound-responsive genes [43] , [44] . Members of the ERF family, such as ERF1 , act as integrators of JA and ethylene signalling in the ethylene/JA-dependent defence response [45] . The members of WRKY family, such as WRKY18 , regulate JA-responsive gene expression [45] , [46] . The JA-inducible transcription factors also include MYB family members, such as MYB24 (refs 35 , 45 , 47 ). Most of these JA-inducible transcription factors act in wound or defence signalling. However, a few JA-responsive transcription factors have been reported to be involved in root development. In this study, we revealed the function of ERF109 in LR formation. ERF109 encodes a member of the B-3 group of the ERF/AP2 transcription factor superfamily with a wide variety of functions in plant growth and development as well as environmental signal transduction [48] . Alignment of the deduced ERF109 protein sequence showed that it has low homology with other members of the superfamily and only limited homology within the AP2 domain, suggesting that ERF109 may have a unique role(s) without genetic redundancy to other ERF family members. Indeed, we have shown that ERF109 -mediated cross-talk of JA signalling and auxin to regulate LR formation by directly activating the auxin biosynthesis genes ASA1 and YUC2 . Despite that several transcription factors can regulate YUC gene expression to affect certain developmental processes [49] , JA-inducible transcription factors-mediated YUC expression is yet to be reported. The transcription factors that regulate ASA1 have not been identified, except for MYB34 / altered tryptophan regulation 1 ( ATR1 ) that activates tryptophan gene expression in Arabidopsis [50] . Taken together, our finding that YUC2 and ASA1 are regulated by ERF109 to affect root development was unexpected. The transcript levels of ASA1 and YUC2 were reduced in erf109 mutants compared with wild type ( Fig. 6a ). Reporter gene analyses also showed slight differences in expression levels of ASA1 and YUC2 between wild type and erf109 ( Fig. 7 ). Furthermore, the auxin level of erf109 plants was reduced ( Figs 4a and 5 ). In addition, ERF109 , ASA1 and YUC2 shared similar expression patterns ( Figs 1 and 7 and Supplementary Fig. 2 ). We provide multiple lines of supporting evidence including yeast-one-hybrid, EMSA and ChIP assays, as well as the genetic analysis that established the interaction between ERF109 and the promoters of both ASA1 and YUC2 genes ( Figs 6 and 7 ). The native promoter of ERF109 was initially used for ChIP assay without success, which was probably due to low expression level of ERF109 , and has been similarly noted for other transcription factors with low expression [51] . However, when we used a stronger promoter, the results showed that ASA1 and YUC2 were targets of ERF109. The erf109 mutant did not show a significant phenotype of root architecture, which may be explained as follows. First, ERF109 had very low expression in root tissue under normal growth conditions, which may reflect the less important role of JA signalling in root development in the absence of environmental stress and the specificity ERF109 for JA signalling in root development. Second, although ERF109 is able to change the auxin content within the root to affect root architecture, the auxin biosynthesis process is a complex metabolic network with multiple biosynthetic routes, and auxin biosynthesis is regulated by many genes with a high level of functional redundancy. Therefore, elimination of ERF109 may have minimally impacted auxin biosynthesis and root development. As shown in Fig. 2a,b , 5-day-old erf109 seedlings had fewer LRP per unit root length than wild type under control conditions, which implies that LRP initiation was either delayed or reduced. However, the lower number of LRP was not reflected in a significant difference in the observed number of LRs ( Fig. 2g and Supplementary Fig. 7a ). We believe that the lack of a significant difference in the number of LRs in our assays may be due to the developmental time lag between LRP formation and LR emergence. Assuming a similar rate of LR emergence, we believe that there was insufficient time in our seedling growth assays for the small difference in the number of LRP to cause a significant difference in the number of LRs. ERF109 overexpression lines had elevated IAA levels in both shoot and root tissues in comparison to wild type ( Figs 4a and 5 ), whereas the expression levels of IAA14 and IAA19 were lower in the shoot tissues ( Fig. 4b,c ). AUX/IAA s genes are auxin-inducible and the response of most AUX/IAAs to IAA is rapid, tissue-specific and dose dependent [52] . In this situation, however, the constitutively elevated IAA levels in ERF109 overexpressors may have inhibited steady-state mRNA accumulation of AUX/IAAs resulting in a different response to what is commonly observed from short-term exogenous IAA treatments. The reduction in LR formation in asa1 is much larger than the reduction in erf109 under MeJA treatment ( Supplementary Fig. 7 ). ASA1 is a downstream target of ERF109. The expression of ASA1 was downregulated in erf109 ( Fig. 6a ) while it was null in asa1 (CS16398) mutant ( Supplementary Fig. 6j ). A higher level of ASA1 expression in erf109 would contribute to the lower reduction in LR formation compared with that in asa1 mutant. In addition, other molecular mechanisms may also be involved in transcriptional regulation of ASA1 and the response of ASA1 to JA. Reduced LR formation in erf109 mutants in response to salt stress suggests that ERF109 has a function in salt-induced LR development ( Supplementary Fig. 8 ). In addition, the weak response of ERF109 to SA and ACC indicates that ERF109 may have a part in cross-talk between SA and IAA, as well as between ethylene and IAA pathways. We also analysed all possible JA-responsive elements in the promoters of ASA1 and YUC2 to identify other transcription factors that may regulate the expression of ASA1 and YUC2 , and many JA-responsive elements were identified. In the YUC2 promoter, one T/G-box (5′- AACGTG -3′), close to the GCC-box, was found. The result implies that there may be other transcription factor(s) involved in the expression of YUC2 in response to JA. In addition, several 5′- GAGTA -3′ motifs were found in both ASA1 and YUC2 promoters. Whether 5′- GAGTA -3′ motifs function in the JA-responsive process is worthy of further study. The identification of several JA-responsive elements in ASA1 and YUC2 promoters further indicate the complexity of interplay of JA and auxin and the important role of ERF109 in mediating JA signals and auxin biosynthesis genes. JA is endogenously produced in response to a variety of environmental stresses and plants adjust accordingly to activate defence responses and modify development processes for survival. In regulation of root development, JA signalling apparently converges with auxin signalling, the major signalling pathway governing root development [49] . Recent research showed that ASA1 and YUCCA were involved in the root response to MeJA treatment [26] . Our results demonstrate that ERF109 acts as an important converging point between JA and auxin signalling pathways by integrating JA signalling into auxin biosynthesis to regulate LR formation. On the basis of our results of auxin accumulation ( Figs 5 and 7e–g ) and no detectable expression of ERF109 in primary root tip ( Fig. 1d,k ), it is possible that ERF109 may affect auxin transport. As a transcription factor, ERF109 is capable of regulating a suite of target genes. It is possible that some target genes fall into the category of auxin transport. Future transcriptome comparison analyses should help to resolve this. Plant materials and growth conditions The wild type used in our study was Arabidopsis thaliana ecotype Columbia-0 (Col-0). A homozygous erf109 loss-function mutant was identified from Salk_150614, which was ordered from Arabidopsis Biological Resource Center. The ERF109pro-GUS , 35S- ERF109 - GFP , 35S- ERF109 and 35S-HA- ERF109 constructs were transformed into Col-0 by Agrobacterium tumefaciens -mediated transformation using strain C58C1. For ERF109pro-GUS , the promoter of ERF109 was amplified and cloned into pDONR207 with the primers GUS/ ERF109 P1 and GUS/ ERF109 P2 ( Supplementary Table 1 ), and subsequently shuttled it into the pCB308R vector to construct the GUS fusion vector. For 35S- ERF109-GFP used in the transient expression assay, the ERF109 -coding region was amplified and cloned into pCB2008E vector to construct the GFP fusion vector with the primers 8E/ERF109 P1 and 8E/ERF109 P2. To obtain 35S- ERF109-GFP transgenic plants, the ERF109 -coding region was amplified and cloned into pDONR207 with primers pGWB5/ERF109 P1 and pGWB5/ERF109 P2, and subsequently shuttled it into pGWB5 vector. For 35S- ERF109 , the ERF109 -coding region was amplified and cloned into pDONR207 with primers pCB2004/ ERF109 P1 and pCB2004/ ERF109 P2 and subsequently shuttled it into pCB2004 vector. To make the 35S-HA- ERF109 construct, which was used for function complementation and ChIP assays, the ERF109 -coding region was amplified and cloned into pDONR207 with the primers HA-ERF109 P1 and HA-ERF109 P2, and subsequently shuttled it into pCB2004 vector. The plant materials DR5-GUS [29] , YUC2pro-GUS [29] and ASA1pro-GUS [28] were used as female parents in genetic analysis, while erf109 , Col-0 and 35S- ERF109 were used as male parents. Arabidopsis seeds were surface sterilized for 10 min in 10% bleach and washed five times at least with sterile water. Plant seeds were kept at 4 °C for 2 days in darkness before germination on horizontal agar plates containing solid Murashige and Skoog (MS) medium with 1% (w/v) sucrose at 22 °C under 16-h light/8-h dark cycles. For analysis of PR length and LR number, 3-day-old seedlings were transferred to MS solid mediums without or with MeJA and grown vertically. The PR length of seedlings grown on medium containing the indicated concentrations of MeJA was measured and the number of LR were counted at the indicated time points. For the detection of transcript level of ERF109 under different hormone and stress treatments, the seedlings were grown on MS medium vertically at first. Then, the 7-day-old or 14-day-old seedlings were transferred to MS medium without (control) or with different hormones or compounds for 0.5 h before RNA extraction or GUS staining. Agrobacterium -mediated transformation of Arabidopsis The constructs were electroporated into Agrobacterium tumefaciens C58C1 and transferred into Arabidopsis using the floral-dip method [53] . Agrobacterium cells containing the appropriate construct were collected by centrifugation. Agrobacterium cells were resuspended using 5% (w/v) sucrose solution until the OD 600 of Agrobacterium cell suspension was 0.8. Silwet L-77, as a strong surfactant, was added to the sucrose solution to obtain a final concentration of 0.05% (v/v). Agrobacterium cell suspension was transferred to the glass dish. Developing Arabidopsis inflorescences were dipped into Agrobacterium cell suspension for about 10 s. The transformed plants were grown in darkness horizontally for 16–24 h. The seeds of treated plants were harvested after Agrobacterium -mediated transformation. The seedlings of transformants were obtained by glufosinate or kanamycin screening. Subcellular localization assay For transient expression assay, the ERF109 -coding region was amplified and cloned into the vector pCB2008E to construct the GFP fusion vector [54] . The inserted sequence was confirmed by sequencing. Then the construct was delivered into the onion epidermal cells via microprojectile bombardment of particle gun. The ERF109 -coding region was also cloned into pGWB5 and the construct was transferred into Col-0 to create transgenic plants. The fluorescence of GFP in onion epidermal cells and the root tissues of transgenic plants were observed under a fluorescence microscope (ZEISS Axio skop2 plus). Analysis of GUS activity The promoter of ERF109 was amplified and cloned into pCB308R (ref. 54 ). Then the construct was transferred into Col-0. Histochemical staining for GUS activity in Arabidopsis was performed using the T2 population [55] . The Arabidopsis seedlings or various tissues were incubated in GUS staining solution containing 0.5 mg ml −1 5-bromo-4-chloro-3-indolyl-b-D-glucuronide cyclohexylamine salt (X-Gluc), 0.1 M sodium phosphate buffer (pH 7.0), 0.5 mM potassium ferricyanide, 0.5 mM potassium ferrocyanide and 0.1% Triton X-100 at 37 °C. Experimental materials were subsequently de-stained and stored in 70% ethanol. The results were observed using a light microscope with a camera (HiROX). Gene expression analysis Total RNA was isolated from various tissues as indicated by the TRIZOL reagent (Invitrogen). The reverse transcription reaction, which was used as template for PCR amplification, was carried out with Prime Script RT reagent Kit (TaKaRa). For RT–PCR analysis, the PCR products were examined on a 1 or 2% agarose gel stained with ethidium bromide. For quantitative RT–PCR analysis, PCR was carried out on a Step One Real-Time PCR system (Applied Biosystems) with the SYBR green (SYBR Premix Ex Taq II, TaKaRa). The transcript levels of target genes were examined using specific primers ( Supplementary Table 1 ). Ubiquitin5 ( UBQ5 , At3g62250) was used as the internal control. Identification of erf109 and transgenic plants of ERF109 Homozygous T-DNA insertion mutants of Salk_150614 were identified using genomic PCR with specific primers and the T-DNA primer LBb1 ( Supplementary Table 1 ) [56] . RT–PCR and quantitative RT–PCR were performed to confirm the results of genomic PCR screen with specific primers ( Supplementary Table 1 ). 35S- ERF109 and FC line were obtained by glufosinate screening and then they were identified by quantitative RT–PCR. Free IAA measurement Free IAA measurement of shoot tissues and root tissues of Col-0, erf109 and 35S- ERF109 seedlings. The Arabidopsis seedlings of Col-0, erf109 and 35S- ERF109 were grown on MS medium containing 1% sucrose. Two-week-old seedlings were divided into shoot tissues and root tissues. Each plant tissue was collected, quickly frozen in liquid nitrogen and ground into a fine powder (200 mg). 2 H-IAA (CDN isotopes) was used as internal standard. Shoot and root tissues were homogenized and extracted for 24 h in methanol containing internal standard. Purification was performed using Oasis Max solid phase extract cartridge (Waters) after centrifugation. IAA measurement was carried out with a liquid chromatography–tandem mass spectrometry system consisted of an Acquity Ultra Performance Liquid Chromatography (Acquity UPLC; Waters) and a triple quadruple tandem mass spectrometer (QTRAP 5500; AB SCIEX) [57] . Yeast-one-hybrid assay Yeast-one-hybrid assay is a powerful technique to rapidly test the interaction between a transcription factor and a regulatory DNA sequence specifically bound by the transcription factor. It was performed using pAD-GAL4-2.1 and the reporter plasmid pHIS2 (ref. 58 ). Briefly, three copies of GCC-box element in tandem repeat were cloned into the reporter plasmid pHIS2. The AtERF109 gene was cloned into the plasmid pAD-GAL4-2.1 to produce the effector plasmid pAD/AtERF109. The reporter and effector plasmids were introduced into yeast cells. The transformants were observed for their growth on SD/-Trp-Leu-His medium or this medium plus 3-aminotriazole (3-AT) following the instruction of the BD Matchmaker Library Construction & Screening Kits ( www.bdbiosciences.com ). To obtain pAD/ERF109 plasmid, the ERF109 -coding region was amplified and cloned into the pAD-GAL4-2.1 vector (AD vector) using Bam HI and Xba I sites with the primers Y1H ERF109 P1 and Y1H ERF109 P2. In pAD/ERF109 plasmid, the ERF109 -coding region was translationally fused to the GAL4-AD domain to express fusion protein for DNA binding in yeast-one-hybrid assay. Then, three pairs of sequences containing GCC-boxes were synthesized with cohesive ends (Sangon of Shanghai, China) ( Supplementary Table 1 ). Each pair of these sequences was annealed and ligated into the Sac I and Mlu I sites of the nutritional reporter plasmid pHIS2 (BD vector). The inserted sequences were confirmed by sequencing. The pAD and pHIS2 empty vector were used as negative control. Different combinations of plasmids were co-transformed into yeast strain Y187 competent cells. Yeast cells were grown on synthetic defined (SD)/-Trp-Leu medium for 3 days at 30°C. Then, yeast cells without or with different dilutions (1:10, 1:100 and 1:1,000) were transferred to SD/-Trp-Leu medium and SD/-Trp-Leu-His medium with 10 mM 3-aminotriazole (3-AT, Sigma), respectively. The yeast cell containing pAD/ERF109 and pHIS2/ cis -element were grown normally on SD/-Trp-Leu-His medium with 10 mM 3-AT, which indicated the interaction between ERF109 and the corresponding cis -element. Identification of JA-responsive elements JA-responsive elements in ASA1 and YUC2 promoters were screened on the basis of the sequence of G-Box (5′- CACGTGG -3′), which can be bound by basic Helix-Loop-Helix (bHLH) transcription factors [59] , [60] ; the hexamer sequence (5′- TGACGT -3′) (ref. 61 ); the JA- and elicitor-responsive element (JERE) [62] ; JASE1 (5′- CGTCAATGAA -3′) and JASE2 (5′- CATACGTCGTCAA -3′) (ref. 63 ); the T/G-box (5′- AACGTG -3′) and GCC-Box [64] , [65] ; a duplicated 5′- GAGTA -3′ motif [66] ; and other JA-responsive motifs reported [67] , [68] . EMSA assay The GST–ERF109 fusion protein was expressed in E. coli strain Rosseta2. 30bp free probes covering GCC-boxes, unlabelled probes (competitor) and mutated probes (non-competitor) carrying 6 bp mutation at GCC-boxes were commercially synthesized (Sangon) as single-stranded (ss) DNA ( Supplementary Table 1 ). Free probes were synthesized and labelled with Digoxigenin (DIG) at the 5′ end. In the mutated probes, the sequence 5′- CATTGA -3′ replaced the core sequence of GCC-box (5′- GCCGCC -3′). Equal amounts of complementary ssDNA were mixed, 95 °C for 5 min and slowly cooled down to 25 °C. EMSA was performed using a DIG Gel Shift Kit, 2nd Generation (Roche). DIG-labelled probes were incubated in 5 × binding buffer (100 mM Hepes, pH 7.6, 5 mM EDTA, 50 mM (NH 4 ) 2 SO 4 , 5 mM DTT, 1% (w/v) Tween 20, 150 mM KCl) with or without GST–ERF109 at room temperature for 20 min. For competition experiments, different amounts of unlabelled and mutated probes were added to the binding reaction. Loading buffer (5 × ) was then added to the binding reaction. Each reaction was loaded on a 4.5% native polyacrylamide gel in 0.5 × TBE buffer. The results were detected using a CCD camera system (Image Quant LAS 4000). ChIP assay Ten-day-old 35S-HA- ERF109 transgenic seedlings and anti-HA antibodies (1:100 for ChIP assay, HA-Tag, 26D11, Mouse mAb, M20003, Abmart, Shanghai, China) were used for ChIP experiments [69] . Briefly, the transgenic seedlings were ground into a fine powder with liquid nitrogen and resuspended in nuclei isolation buffer. The nucleus were then collected by centrifugation and resuspended with nuclei lysis buffer. The resuspended chromatin was sonicated to fragments with various sizes (250 bp–1 kb) subsequently. HA-ERF109 was precipitated from input DNA with anti-HA antibodies or without any antibodies. Protein A agarose beads (Millipore, USA) were added into the incubation mixture for additional 2 h at 4 °C. The immune complexes were eluted from the washed protein A beads. The DNA was purified with phenol/chloroform (1:1, v/v) and precipitated. The purified DNA and input DNA were used as templates. The enrichments of DNA fragments were determined by RT–PCR and quantitative RT–PCR with specific primers ( Supplementary Table 1 ; ref. 70 ). Genetic analysis Crosses were generated by transferring pollen from mature anthers of male parent to the stigmas of previously emasculated flowers of female parent. How to cite this article : Cai, X.-T. et al . Arabidopsis ERF109 mediates cross-talk between jasmonic acid and auxin biosynthesis during lateral root formation. Nat. Commun. 5:5833 doi: 10.1038/ncomms6833 (2014).